Anion stabilisedhypercloso-hexaalane Al6H6 Boron hydride clusters are an extremely diverse compound class, which are of enormous importance to many areas of chemistry. Despite this, stable aluminium hydride analogues of these species have remained staunchly elusive to synthetic chemists. Here, we report that reductions of an amidinato-aluminium(III) hydride complex with magnesium(I) dimers lead to unprecedented examples of stable aluminium(I) hydride complexes, [( Ar Nacnac)Mg] 2 [Al 6 H 6 (Fiso) 2 ] ( Ar Nacnac = [HC(MeCNAr) 2 ] − , Ar = C 6 H 2 Me 3 -2,4,6 Mes; C 6 H 3 Et 2 -2,6 Dep or C 6 H 3 Me 2 -2,6 Xyl; Fiso = [HC(NDip) 2 ] − , Dip = C 6 H 3 Pr i 2 -2,6), which crystallographic and computational studies show to possess near neutral, octahedral hypercloso -hexaalane, Al 6 H 6 , cluster cores. The electronically delocalised skeletal bonding in these species is compared to that in the classical borane, [B 6 H 6 ] 2− . Thus, the chemistry of classical polyhedral boranes is extended to stable aluminium hydride clusters for the first time. The binary hydrides of boron, i.e. boranes (typically [B x H y ] z − , x ≤ y , z = 0–2), are of enormous importance to chemistry from both fundamental and applications standpoints. The vast majority of these species are low oxidation state boron cluster compounds, which exhibit an enormous array of structural types [1] . The understanding of the structures of such clusters required the early development of revolutionary theories on chemical bonding (e.g. Wade–Mingos rules for electron counting) [2] , [3] , which ultimately led to boranes finding applications in areas as diverse as synthesis [4] , rocket fuel technology [5] and medical science [6] . It is remarkable that aluminium, boron’s neighbour in group 13, does not form any isolable hydride cluster compounds, or indeed many binary hydride compounds at all, e.g. AlH 3 , H 2 Al(μ-H) 2 AlH 2 and [AlH 4 ] − [7] . With that said, a handful of transient, low oxidation state alane cluster compounds have been studied in the gas phase, and some, e.g. Al 4 H 6 , have been shown to have fleeting stability [8] , [9] , [10] , [11] . Given that numerous ligand substituted, metalloid aluminium cluster compounds, e.g. [Al 77 {N(SiMe 3 )} 20 ] 2− , have been reported to be stable at, or close to, room temperature [12] , [13] , it seemed that related low-valent aluminium hydride clusters might be ultimately accessible under the right preparative conditions. As a prelude to realising this goal, we have synthesised the first stable binary low oxidation state aluminium hydride fragments, viz. [Al 2 H 6 ] 2− and Lewis base stabilised Al 2 H 4 , by reduction of aluminium(III) hydride precursors with magnesium(I) dimers [14] , [15] . Here, we report that related reductions of an amidinato-aluminium(III) hydride complex lead to unprecedented examples of stable aluminium(I) hydride complexes, [( Ar Nacnac)Mg] 2 [Al 6 H 6 (Fiso) 2 ] ( Ar Nacnac = [HC(MeCNAr) 2 ] − , Ar = C 6 H 2 Me 3 -2,4,6 Mes; C 6 H 3 Et 2 -2,6 Dep or C 6 H 3 Me 2 -2,6 Xyl; Fiso = [HC(NDip) 2 ] − , Dip = C 6 H 3 Pr i 2 -2,6), which possess near neutral hypercloso -hexaalane, Al 6 H 6 , cluster cores. Thus, this work represents a unique extension of the chemistry of classical polyhedral boranes to that of their alane analogues. Synthetic and spectroscopic studies Treatment of benzene, toluene, cyclohexane or hexane solutions of the formamidinato-aluminium(III) hydride complex, [{(μ- N,N -Fiso)Al(H)(μ-H)} 2 ] [16] , with 1.2–2.0 equivalents of β-diketiminato ligated magnesium(I) dimers, [{( Ar Nacnac)Mg} 2 ] (Ar = Mes, Dep or Xyl) [17] , [18] , [19] (see Supplementary Materials and Supplementary Figs. 1 – 5 ), at elevated temperatures (typically 60–80 °C) reproducibly afforded low yields (ca. 5–20%) of the deep red crystalline aluminium(I) hydride cluster compounds 1 (Fig. 1 ), upon cooling the reaction solutions to ambient temperature. On several occasions, a number of low yielding colourless crystalline by-products were isolated from the reaction mixtures, including [(Fiso)Mg( Dep Nacnac)], [(Fiso) 2 AlH] [16] , [{( Mes Nacnac)Mg(μ-H)} 2 ] [15] and the dialanate salt, [{( Mes Nacnac)Mg} 2 (μ-H)] 2 [H 3 Al–AlH 3 ] [14] (see Supplementary Methods and Supplementary Figs. 6 – 9 ). The nature of these by-products suggests that the reductive mechanism for the formation of 1 could involve several intermediates and/or could compete with side reactions. In order to assess these possibilities, reactions that gave 1 at 70 °C were followed by 1 H NMR spectroscopy. This revealed complex mixtures of products after several minutes heating, of which [(Fiso)Mg(Nacnac)] was identified in significant quantities (Supplementary Fig. 10 ). Definitive identification of products, other than those which were later isolated as crystalline solids, was not possible, and the mechanism of formation of 1 is not certain at this time. Fig. 1 Formation of compounds 1 (Mes = C 6 H 2 Me 3 -2,4,6; Dep = C 6 H 3 Et 2 -2,6; Xyl = C 6 H 3 Me 2 -2,6). The compounds 1 are prepared by reduction of [{(μ- N,N -Fiso)Al(H)(μ-H)} 2 ] with magnesium(I) dimers Full size image To the best of our knowledge compounds 1 represent the first examples of isolated aluminium(I) hydride complexes, though mononuclear examples have recently been tentatively proposed as unstable intermediates in solution-based reactions [20] . The cluster compounds have negligible solubility in common deuterated solvents once crystallised, so no meaningful solution state spectroscopic data could be acquired for them. The most relevant solid state spectroscopic data (Supplementary Figs. 11 , 12 ) for the compounds come from their infrared spectra, which exhibit single bands in the characteristic region for terminal Al–H stretching modes [7] (e.g. 1a : ν = 1798 cm −1 ). In addition, stronger bands are seen at lower wavenumber (e.g. 1a : ν = 1648 cm −1 ) that possibly arise from a weakly bridging Al–H···Mg stretching mode, though these bands overlap with ligand stretching absorptions (see below). Noteworthy is the fact that the band at ν = 1798 cm −1 observed for 1a is completely absent in the infrared spectrum of its hexa-deuteride analogue, 1a-D , which was prepared by magnesium(I) reduction of [{(μ- N,N -Fiso)Al(D)(μ-D)} 2 ]. The Al-D stretching band for 1a-D should occur at ca. 1270 cm −1 , but this is likely masked by strong ligand stretching modes in that region (Supplementary Fig. 12 ). Crystallographic studies All complexes 1 were crystallographically characterised and found to be isostructural, so only the molecular structure of 1a is depicted in Fig. 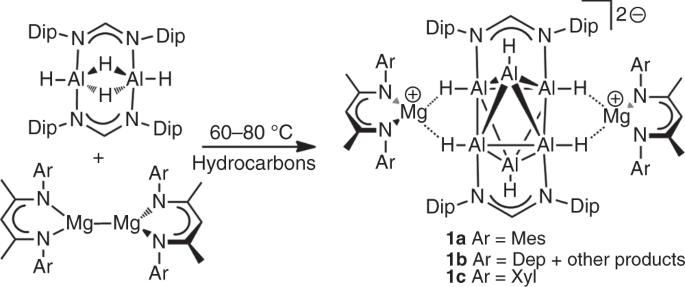Fig. 1 Formation of compounds1(Mes = C6H2Me3-2,4,6; Dep = C6H3Et2-2,6; Xyl = C6H3Me2-2,6). The compounds1are prepared by reduction of [{(μ-N,N-Fiso)Al(H)(μ-H)}2] with magnesium(I) dimers 2 (see Supplementary Methods, Supplementary Table 1 and Supplementary Figures 13 and 14 ). The hydride ligands of each cluster were located from difference maps and freely refined. A neutron diffraction study was also carried out on compound 1a , which unambiguously confirmed the presence and connectivity of the six hydride ligands, and the absence of any other terminal, bridging or interstitial hydrides within the cluster core (see Supplementary Methods and Supplementary Figs. 15 , 16 ). The compounds can be considered as having near neutral, distorted octahedral Al 6 H 6 cores, opposing equatorial sides of which are coordinated by bridging, electronically delocalised formamidinate ligands. The remaining equatorial sides of the octahedron are bridged by [( Mes Nacnac)Mg] + cations, which have weak interactions with the two hydride ligands that project from each side. Terminal hydride ligands coordinate to the apical aluminium centres of the cluster core, though these are slightly offset from the vector passing through the two aluminium centres to which they are coordinated, presumably for steric reasons. All of the Al–Al distances within the Al 6 core lie in the known range for such bonds (mean: 2.72(12) Å, search of the Cambridge Crystallographic Database, February 2018), though the equatorial Al–Al distances (2.701(2) Å and 2.826(2) Å) are significantly longer than those between all axial and equatorial aluminium centres (2.631(2)–2.691(2) Å). The shorter of the equatorial Al–Al interactions are, not surprisingly, those which are bridged by the formamidinate ligands. Fig. 2 Molecular structure of 1a . Hydrogen atoms, except hydrides, omitted. Ellipsoids shown at the 20% probability level, except aryl substituents, which are shown as wire frame. Selected bond lengths (Å): Al(1)–Al(2) 2.6317(15), Al(1)–Al(3) 2.6340(17), Al(1)–Al(2)′ 2.6472(15), Al(1)–Al(3)′ 2.6907(18), Al(2)–Al(3) 2.701(2), Al(2)–Al(3)′ 2.8257(14), Al(3)–N(2) 1.950(3), Al(2)–N(1) 1.925(3), Al(1)–H(1) 1.52(3), Al(2)–H(2) 1.55(3), Al(3)–H(3) 1.57(3), Mg(1)–H(2) 1.96(3), Mg(1)–H(3)′ 1.98(3). Symmetry operation: − x + 2, − y + 1, − z Full size image Electronic structure and computational studies The neutral distorted, octahedral Al 6 H 6 cluster cores of 1 somewhat resemble the structure of the classical polyhedral borane, closo -[B 6 H 6 ] 2− [1] , despite their aforementioned elongated equatorial Al–Al interactions. This is intriguing as Al 6 H 6 can be viewed as having 12 (i.e. 2 n ) valence electrons (i.e. 2 from each Al vertex) contributing to the skeletal Al–Al bonding of the cluster core. As such, it would be expected to have a more unsymmetrical, capped structure than the 14 skeletal valence electron (2 n + 2) closo -[B 6 H 6 ] 2− , according to Wade–Mingos rules [2] , [3] . Indeed, computational studies have predicted a number of more open and unsymmetrical structures for Al 6 H 6 [21] , [22] , which are close in energy. Of course, in 1 the distorted octahedral geometry of this fragment is likely enforced by coordination to the amidinate ligands, which computational studies suggest do not add to the skeletal electron count (see below). For sake of comparison, isoelectronic B 6 H 6 and Ga 6 H 6 , which have not been isolated experimentally, have been predicted to have capped trigonal bipyramidal hypercloso -structures, with all hydrides terminal [23] , [24] . Also worthy of mention are several ligand substituted analogues of Al 6 H 6 , e.g. B 6 (NMe 2 ) 6 [25] and Ga 6 {SiMe(SiMe 3 ) 2 } 6 [24] , which possess distorted octahedral structures with several elongated E–E bonds, not dissimilar to the situation in 1 . In the case of Ga 6 {SiMe(SiMe 3 ) 2 } 6 , calculations on the model compound Ga 6 H 6 suggest that this can be attributed to a Jahn–Teller distortion arising from loss of degeneracy of the t 2g HOMOs of closo -[Ga 6 H 6 ] 2− upon removal of two electrons from that dianion [24] . In order to shed light on the nature of the bonding in the Al 6 H 6 core of 1 , DFT calculations (theory level: RI-BP86/def2-TZVPP) were carried out on a cut-down model of the cluster compounds, viz. [( Me Nacnac)Mg] 2 [Al 6 H 6 ( H Fiso) 2 ] 1′ ( Me Nacnac = [HC(MeCNMe) 2 ] − , H Fiso = [HC(NH) 2 ] − ) (Supplementary Methods). The geometry of the complex (Supplementary Fig. 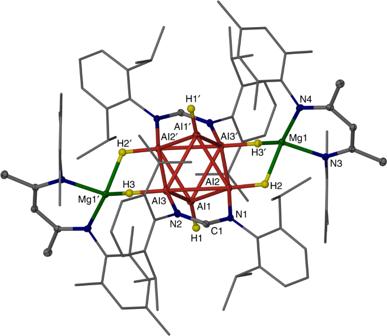Fig. 2 Molecular structure of1a. Hydrogen atoms, except hydrides, omitted. Ellipsoids shown at the 20% probability level, except aryl substituents, which are shown as wire frame. Selected bond lengths (Å): Al(1)–Al(2) 2.6317(15), Al(1)–Al(3) 2.6340(17), Al(1)–Al(2)′ 2.6472(15), Al(1)–Al(3)′ 2.6907(18), Al(2)–Al(3) 2.701(2), Al(2)–Al(3)′ 2.8257(14), Al(3)–N(2) 1.950(3), Al(2)–N(1) 1.925(3), Al(1)–H(1) 1.52(3), Al(2)–H(2) 1.55(3), Al(3)–H(3) 1.57(3), Mg(1)–H(2) 1.96(3), Mg(1)–H(3)′ 1.98(3). Symmetry operation: −x+ 2, −y+ 1, −z 7 and Supplementary Table 2 ) optimised to be similar to those of 1 , including a distorted octahedral Al 6 H 6 core with somewhat shorter Al ax –Al eq bonds (2.650–2.668 Å) than Al eq –Al eq distances (2.718–2.819 Å). 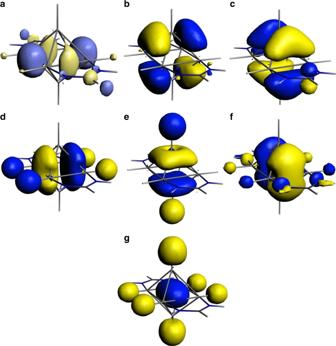Fig. 3 Representations of the aluminium-based MOs of [Al6H6(HFiso)2]2−.aLUMO+7 (5.64 eV),bHOMO (3.42 eV),cHOMO-1 (3.30 eV),dHOMO-2 (1.96 eV),eHOMO-3 (1.84 eV),fHOMO-4 (1.70 eV),gHOMO-9 (−0.01 eV) Reassuringly, the calculated infrared spectrum of 1′ (Supplementary Table 3 ) exhibits terminal and bridging Al–H stretching bands ( ν = 1797 cm −1 (m) and 1649 cm −1 (s) respectively) that are very close to the experimental values for 1a , thus supporting the use of 1′ as a model for 1 . The charges on the whole Al 6 H 6 fragment (−0.67), both H Fiso ligands (−1.10) and both ( Me Nacnac)Mg fragments (+1.76) (Supplementary Table 4 ), indicate that 1′ is best viewed as an anion coordinated, near neutral hypercloso -Al 6 H 6 cluster, having weak hydride bridges to [( Me Nacnac)Mg] + cationic units. The calculated Wiberg bond indices (WBI) for the Al ax –Al eq bonds (0.63–0.66) (Supplementary Table 5 ) are suggestive of relatively strong bonding interactions, while the WBIs for the Al eq -Al eq interactions are much smaller (0.23–0.31). In line with this result is the fact that no bond critical points were found between the equatorial aluminium centres (Supplementary Fig. 8 ). Calculations on the [Al 6 H 6 ( H Fiso) 2 ] 2− dianion, in the absence of the [( Me Nacnac)Mg] + cations, showed this fragment to be stable, with a geometry similar to that in the full contact ion compound (Supplementary Fig. 17 and Supplementary Table 2 ). This, combined with the fact that the uncoordinated Al 6 H 6 octahedral unit was calculated to be an unstable entity in the electronic singlet state, confirms that the hypercloso -Al 6 H 6 moiety of 1′ is stabilised by coordination to the H Fiso anions. The electronic structure of the [Al 6 H 6 ( H Fiso) 2 ] 2− dianion was calculated and found to be similar to that of the full contact ion compound (Supplementary Figs. 19 – 21 ), so only the former is displayed in Fig. 3 . There are seven Al-based molecular orbitals (MOs) on the dianion, six of which are filled, in line with the view that the cluster is a 12 skeletal valence electron species. None of these MOs are degenerate, but they do closely resemble the seven filled cluster based MOs for closo -[B 6 H 6 ] 2− (triply degenerate t 2g and t 1u orbital sets, and a 1g orbital) [2] , and thus display significant electronic delocalisation over the Al 6 core. The lack of degeneracy of the Al-based MOs of [Al 6 H 6 ( H Fiso) 2 ] 2− arises from the lower symmetry, and lower skeletal electron count, of the dianion relative to those of closo -[B 6 H 6 ] 2− . Interestingly, the LUMO+7 (lower energy empty MOs are ligand based) of [Al 6 H 6 ( H Fiso) 2 ] 2− resembles the degenerate t 2g HOMO of closo -[B 6 H 6 ] 2− which exhibits the most analogous, quasi -equatorial B–B bonding character. This goes a long way to explaining the weak Al eq –Al eq interactions in 1′ . The HOMO and HOMO-1 of [Al 6 H 6 ( H Fiso) 2 ] 2− are reminiscent of the other two t 2g orbitals of closo -[B 6 H 6 ] 2− , while the HOMO-2, HOMO-3 and HOMO-4 show similarities with the t 1u orbitals of the borane. At lower energy is the HOMO-9 which corresponds to the a 1g orbital of closo -[B 6 H 6 ] 2− . No Al-based MO exhibits significant contributions from the H Fiso anions, the lone pairs of which are polarised towards their N -centres, and should therefore not be included in the counting of electrons contributing to Al–Al bonding within the cluster core. This view is supported by results of an energy decomposition analysis of the intrinsic interactions between the Al 6 H 6 core and the amidinate ligands in [Al 6 H 6 ( H Fiso) 2 ] 2− (Supplementary Fig. 22 and Supplementary Table 6 ). Calculations of the NICS values of 1′ at the centre of the Al 6 H 6 core suggest that the cluster exhibits significant 3-dimensional aromaticity (NICS iso = −12.49 ppm, NICS zz = −45.74 ppm) (Supplementary Table 7 ), as is common for polyhedral boranes [1] . Fig. 3 Representations of the aluminium-based MOs of [Al 6 H 6 ( H Fiso) 2 ] 2− . a LUMO+7 (5.64 eV), b HOMO (3.42 eV), c HOMO-1 (3.30 eV), d HOMO-2 (1.96 eV), e HOMO-3 (1.84 eV), f HOMO-4 (1.70 eV), g HOMO-9 (−0.01 eV) Full size image General Experiments were carried out under a dry, oxygen-free dinitrogen atmosphere using Schlenk-line and glove-box techniques. All solvents and reagents were rigorously dried and deoxygenated before use. Compounds were variously characterised by elemental analyses, NMR, FTIR, and Raman spectroscopies, single crystal X-ray diffraction studies, and DFT calculations. Further details are available in Supplementary Methods. Preparation of [( Xyl Nacnac)MgI(OEt 2 )] A freshly prepared solution of MeMgI (28.4 mmol) in diethyl ether (80 mL) was added over 20 min to a stirred solution of Xyl NacnacH [26] (8.08 g, 26.4 mmol) in diethyl ether (100 mL) at −20°C, yielding a colourless precipitate. The suspension was warmed to room temperature and stirred for 1 h after which time the precipitate of the title compound was collected by filtration. The supernatant solution was concentrated to ca. 40 mL and cooled to −30 °C to afford a second crop (12.86 g, 90%). M.P. 195–197 °C (decomp. ); 1 H NMR (400 MHz, 298 K, C 6 D 6 ) δ = 0.44 (br, 6H; OCH 2 C H 3 ), 1.54 (s, 6H; NCC H 3 ), 2.07 (br, 6H; ortho -C H 3 ), 2.64 (br, 6H; ortho -C H 3 ), 3.11 (br, 4H; OC H 2 CH 3 ), 4.86 (s, 1H; C H ), 6.75–7.15 (m, 6H; Ar- H ); 13 C{ 1 H} NMR (100 MHz, 298 K, C 6 D 6 ) δ = 13.0 (NC C H 3 ), 18.7 ( ortho - C H 3 ), 21.1 ( ortho - C H 3 ), 23.4 (OCH 2 C H 3 ), 65.9 (O C H 2 CH 3 ), 95.3 ( C H), 124.7, 129.6, 131.5, 147.7 (Ar- C ), 168.8 (N C CH 3 ); MS (EI 70 eV), m / z (%): 457.1 (MH + -OEt 2 , 5), 306.4 ( Xyl NacnacH + , 100); IR (Nujol) ν (cm −1 ): 1518s, 1262m, 1215w, 1197m,1185m, 1148m, 1092m, 1021m, 996m, 857m, 848w, 775s, 758m, 636m. Note: A satisfactory reproducible microanalysis of the compound could not be obtained due to co-crystallisation of the product with small amounts (ca. 3%) of the β-diketimine, Xyl NacnacH, which could not be removed after several recrystallisations. Preparation of [{( Xyl Nacnac)Mg} 2 ] Toluene (80 mL) and diethyl ether (ca. 2 mL) were added to [( Xyl Nacnac)MgI(OEt 2 )] (1.58 g, 2.40 mmol). The resultant solution was rapidly stirred over a sodium mirror (0.70 g, 30.4 mmol) for 5 days to yield a yellow/green suspension. This was filtered, the yellow filtrate concentrated to ca. 20 mL and placed at −30 °C overnight to give yellow crystals of the title compound. A second crop was isolated after further concentration and cooling of the supernatant solution (0.28 g, 29%). M.P. 180–181 °C (decomp. ); 1 H NMR (400 MHz, 298 K, C 6 D 6 ) δ = 1.48 (s, 12H; NCC H 3 ), 1.90 (br. s, 24H; ortho -C H 3 ), 4.76 (s, 2H; C H ), 6.85–7.10 (m, 12H; Ar- H ); 13 C{ 1 H} NMR (100 MHz, 298 K, C 6 D 6 ) δ = 19.2 (NC C H 3 ), 23.1 ( ortho - C H 3 ), 95.3 ( C H), 124.1, 128.4, 131.8, 148.0 (Ar- C ), 166.3 (N C CH 3 ); MS (EI 70 eV), m / z (%): 659.5 (MH + , 10); IR (Nujol) ν (cm −1 ): 1555s, 1520w, 1278m, 1262m, 1182m, 1094m, 1023m, 809w, 762m. Note: A satisfactory reproducible microanalysis of the compound could not be obtained due to co-crystallisation of the product with small amounts (ca. 5%) of the iodide bridged magnesium(II) dimer, [{( Xyl Nacnac)Mg(μ-I)} 2 ], which could not be removed after several recrystallisations. The constitution of this co-crystallised mixture was confirmed by a poor quality crystal structure determination of [{( Xyl Nacnac)Mg} 2 ], details of which are not reported here due to the low quality of the diffraction data. Preparation of [( Mes Nacnac)Mg] 2 [Al 6 H 6 (Fiso) 2 ] ( 1a ) [{(μ- N,N -Fiso)Al(H)(μ-H)} 2 ] [16] (164 mg, 0.21 mmol) was added to a suspension of [{( Mes Nacnac)Mg} 2 ] [27] (300 mg, 0.42 mmol) in benzene (5 mL) in a grease-free Schlenk flask (20 mm diameter). The mixture was heated to 65 °C for 5 min or until a bright red solution formed. Allowing the solution to stand at room temperature for 4 days resulted in the deposition of red crystals of 1a (20 mg, 18% based on aluminium). M.P. > 150 °C (decomp.) 13 C{ 1 H} NMR (75.5 MHz, 298 K, solid state) δ = 17.5, 20.6, 25.4, 27.7, 95.1, 123.8, 129.4, 131.5, 142.1, 146.4, 163.4, 167.4; MS (EI 70 eV), m / z (%): 335.5 ( Mes NacnacH 2 + , 100), 365.5 (FisoH 2 + , 38); MALDI-TOF MS m / z : 335.5 ( Mes NacnacH 2 + ), 357.4 (( Mes Nacnac)Mg + ), 365.5 (FisoH 2 + ), 389.4 ((Fiso)Al–H + ); IR (Nujol) ν (cm −1 ): 1798m (Al–H str. ), 1648s (br, incl. Al–H str. ), 1542vs, 1197m, 1176m, 1146s, 1097s, 1021s, 854s, 803s, 755s; Raman (solid under N 2 , 514 nm excitation, cm −1 ): ν = 3064m, 1352s, 1318m, 522m, 386m. A similar yield of 1a was obtained when the reaction was conducted in cyclohexane (ca. 12 mL). Elemental analysis calculated for C 96 H 134 Al 6 Mg 2 N 8 ·C 6 H 12 : C 72.29%, H 8.68%, N 6.61%; found: C 72.13%, H 8.55%, N 6.54%. Notes: (i) A few crystals of the known magnesium(II) hydride dimer, [{( Mes Nacnac)Mg(μ-H)} 2 ] [15] , the known aluminium(III) hydride, [(Fiso) 2 AlH] [16] , and the new colourless dialanate salt, [{( Mes Nacnac)Mg} 2 (μ-H)] 2 [H 3 Al–AlH 3 ], co-crystallised with 1a from the reaction mixture. All were identified by X-ray crystallography (Supplementary Fig. 9 ). Insufficient amounts of [{( Mes Nacnac)Mg} 2 (μ-H)] 2 [H 3 Al–AlH 3 ] were obtained to allow spectroscopic characterisation, but it is noteworthy that the 2,6-diethylphenyl substituted analogue of the compound, [{( Dep Nacnac)Mg} 2 (μ-H)] 2 [H 3 Al–AlH 3 ], has been previously reported and fully characterised [14] . (ii) Reproducible low yield syntheses of 1a (typically 5–20%) were achieved under a number of reaction conditions. For example, toluene, hexane, cyclohexane or benzene could be used as the reaction solvent, the reaction temperature was varied from ca. 60–80 °C, the reaction stoichiometry was varied from 1.2:1 to 2:1 ([{( Mes Nacnac)Mg} 2 ]:[{(μ- N,N -Fiso)Al(H)(μ-H)} 2 ]), and the time the reaction mixture was kept at elevated temperature varied from 5 to 25 min. The time required for the reaction depended strongly on the diameter of the reaction flask. (iii) Compound 1a (and 1b-c ) have negligible solubility in common deuterated solvents once crystallised, so no meaningful solution state spectroscopic data could be acquired for them. Attempts to dissolve 1a in d 8 -THF led to decomposition of the compound. (iv) Attempts were made to obtain solution state spectroscopic data on 1a from red reaction solutions before it crystallised from those solutions. NMR spectroscopic data on those solutions showed complex product mixtures (Supplementary Fig. 10 ), while ESI mass spectroscopic analyses of the reaction solutions showed no ion that could be assigned to 1a or its fragmentation products. Preparation of [( Dep Nacnac)Mg] 2 [Al 6 H 6 (Fiso) 2 ] ( 1b ) [{(μ- N,N -Fiso)Al(H)(μ-H)} 2 ] [16] (102 mg, 0.13 mmol) was added to a suspension of [{( Dep Nacnac)Mg} 2 ] [19] (200 mg, 0.26 mmol) in benzene (2 mL) in a grease-free Schlenk flask (20 mm diameter). The mixture was heated to 65 °C for 5 min or until a bright red solution formed. Allowing the solution to stand at room temperature for 4 days resulted in the deposition of deep red crystals of 1b (10 mg, 5% based on aluminium). M.P. > 150 °C (decomp. ); IR (Nujol) ν (cm −1 ): 1834m (Al–H str. ), 1633s (br, incl. Al–H str. ), 1538s, 1366vs, 1338s, 1320s, 1261s, 1232m, 1177s, 1108s, 1023s, 946m, 802s. No solution state spectroscopic data could be obtained for the compound due to its negligible solubility in common organic solvents. A reproducible microanalysis of the compound could not be obtained due it its low yield and the fact that it co-crystallised with the known dialanate salt, [{( Dep Nacnac)Mg} 2 (μ-H)] 2 [H 3 Al–AlH 3 ] [14] , and the new, colourless magnesium(II) complex, [(Fiso)Mg( Dep Nacnac)]. The latter compound was subsequently intentionally synthesised, spectroscopically characterised, and its X-ray crystal structure obtained (Supplementary Figure 8 ). Preparation of [( Xyl Nacnac)Mg] 2 [Al 6 H 6 (Fiso) 2 ] ( 1c ) [{(μ- N,N -Fiso)Al(H)(μ-H)} 2 ] [16] (118 mg, 0.15 mmol) was added to a suspension of [{( Xyl Nacnac)Mg} 2 ] (200 mg, 0.30 mmol) in benzene (3 mL) in a grease-free Schlenk flask (20 mm diameter). The mixture was heated to 65 °C for 5 min or until a bright red solution formed. Allowing the solution to stand at room temperature for 4 days resulted in the deposition of deep red crystals of 1c (10 mg, 4% based on aluminium). M.P. > 150 °C (decomp. ); IR (Nujol) ν (cm −1 ): 1829m (Al–H), 1623m (br incl. Al–H str. ), 1593m, 1543vs, 1336s, 1322s, 1265m, 1257m, 1233m, 1185s, 1096m, 1031m, 951m, 934m, 843m, 802m, 762s, 698m. No solution state spectroscopic data could be obtained for the compound due to its negligible solubility in common organic solvents. A reproducible microanalysis of the compound could not be obtained due it its low yield and the fact that it co-crystallised with colourless crystalline compounds from which it could not be completely separated. Preparation of [( Mes Nacnac)Mg] 2 [Al 6 D 6 (Fiso) 2 ] ( 1a-D ) [{(μ- N,N -Fiso)Al(D)(μ-D)} 2 ] (165 mg, 0.21 mmol), prepared as per the procedure for [{(μ- N,N -Fiso)Al(H)(μ-H)} 2 ] [16] (see Supplementary Methods), was added to a suspension of [{( Mes Nacnac)Mg} 2 ] [27] (300 mg, 0.42 mmol) in benzene (5 mL) in a grease-free Schlenk flask (20 mm diameter). The mixture was heated to 65 °C for 5 min or until a bright red solution formed. Allowing the solution to stand at room temperature for 4 days resulted in the deposition of red crystals of 1a (21 mg, 19% based on aluminium). M.P. > 150 °C (decomp. ); IR (Nujol) ν (cm −1 ): 1665m, 1546s, 1388vs, 1366vs, 1338s, 1259s, 1231m, 1195m, 1146s, 1098s, 1022s, 856m, 803m, 754s, 698s; Raman (solid under N 2 , 514 nm excitation, cm −1 ): ν = 1353s, 1320m, 523w, 445m, 380w. Preparation of [(Fiso)Mg( Dep Nacnac)] This compound was a by-product in the preparation of 1b . It was subsequently intentionally synthesised as follows. Toluene (10 mL) was added to a solid mixture of [{( Dep Nacnac)Mg(μ- n Bu)} 2 ] [19] (0.390 g, 0.440 mmol) and FisoH (0.331 g, 0.907 mmol) at room temperature. The mixture was then stirred for 90 min at 40 °C to afford a colourless solution. The resultant solution was concentrated under reduced pressure to 3 mL, n -hexane (4 mL) was added, and the solution was stored at −30 °C overnight to afford colourless crystals of [(Fiso)Mg( Dep Nacnac)] (0.31 g, 47%). M.P. : gradually softens above 210 °C and takes on a yellow colour above 290 °C; 1 H NMR (300 MHz, C 6 D 6 , 303 K): δ = 1.06 (d, 3 J H,H = 6.9 Hz, 24H; CH(C H 3 ) 2 ), 1.10 (t, 3 J H,H = 7.6 Hz, 12H; CH 2 C H 3 ), 1.53 (s, 6H; NCC H 3 ), 2.55 (dq, 2,3 J H,H = 15.0 Hz, 7.5 Hz, 4H; C H 2 CH 3 ), 2.67 (dq, 2,3 J H,H = 15.0 Hz, 7.5 Hz, 4H; C H 2 CH 3 ), 2.99 (sept, 3 J H,H = 6.9 Hz, 4H; C H (CH 3 ) 2 ), 4.92 (s, 1H; C H ), 6.96–7.10 (m, 12H; Ar- H ), 7.94 (s, 1H; N 2 C H ); 13 C{ 1 H} NMR (75.5 MHz, C 6 D 6 , 303 K): δ = 13.8 (CH 2 C H 3 ), 23.8 (NC C H 3 ), 24.6 ( C H 2 CH 3 ), 25.0 (CH( C H 3 ) 2 ), 28.7 (CH( C H 3 ) 2 ), 96.0 ( C H), 123.6, 123.9, 125.3, 125.9, 137.2, 142.5, 143.8, 147.4 (Ar- C ), 169.9 (N C CH 3 ), 171.5 (N 2 C H); IR (Nujol): ν (cm −1 ) = 1665m, 1595w, 1537s, 1531s, 1505m, 1462s, 1443s, 1390s, 1377s, 1321m, 1274s, 1266s, 1207m, 1181m, 1108m, 1031m, 1018m, 962w, 934m, 854m, 806m, 799m, 755s, 722m; elemental analysis calculated for C 50 H 68 N 4 Mg: C 80.13%, H 9.14%, N 7.48%; found: C 80.03%, H 9.17, N 7.43%. Data availability The X-ray crystallographic coordinates for structures reported in this study have been deposited at the Cambridge Crystallographic Data Centre (CCDC), under deposition numbers 1830325–1830331. These data can be obtained free of charge from The Cambridge Crystallographic Data Centre via www.ccdc.cam.ac.uk/data_request/cif .